Elucidation ofIgH3′ region regulatory role during class switch recombination via germline deletion In mature B cells, class switch recombination (CSR) replaces the expressed constant Cμ gene with a downstream C H gene. How the four transcriptional enhancers of the IgH 3′ regulatory region ( 3′RR ) control CSR remains an open question. We have investigated IgG 1 CSR in 3′RR -deficient mice. Here we show that the 3′RR enhancers target the S γ1 acceptor region (and poorly the S μ donor region) by acting on epigenetic marks, germline transcription, paused RNA Pol II recruitment, R loop formation, AID targeting and double-strand break generation. In contrast, location and diversity of S μ - S γ1 junctions are not affected by deletion of the 3′RR enhancers. Thus, the 3′RR controls the first steps of CSR by priming the S acceptor region but is not implicated in the choice of the end-joining pathway. Lymphopoiesis is coupled with programmed accessibility of Ig genes to transcription and to several major transcription-dependent DNA remodelling events [1] , [2] . Multiple cis -regulatory elements located 5′ and 3′ of constant ( C ) genes control B-cell ontogeny (schematised in the Supplementary Fig. 1a ). Among 5′ elements, the intronic Eμ enhancer is reported as a master control element of V(D)J recombination [3] , [4] . The IgH 3′ regulatory region ( 3′RR ), that encompasses the four transcriptional enhancers hs3a , hs1,2 , hs3b and hs4 , controls μ transcription in mature B-cells [5] , and is the master element controlling conventional class switch recombination (CSR) [6] , [7] and somatic hypermutation (SHM) [8] but without role on V(D)J recombination [9] , [10] . CSR is a cis -deletion or trans -recombination process that allows the C μ gene to be replaced in mice with one of the downstream C γ3 , C γ1 , C γ2b , C γ2a , C ɛ or C α gene. These C genes are preceded by repetitive target sequences for CSR termed switch ( S ) regions. CSR thus usually joins the most 5′ S donor region ( S μ ) and one of the downstream S acceptor regions ( S γ3 , S γ1 , S γ2b , S γ2a , S ɛ or S α ) (schematised in the Supplementary Fig. 1a ). CSR is a complex process involving epigenetic histone modifications for transcriptional accessibility, germline transcription, pausing of RNA Pol II, R loop formation, AID recruitment, AID-induced DNA double-strand breaks (DSBs) and their repair by means of end joining [11] , [12] , [13] , [14] , [15] . CSR uses the classical non-homologous end joining (C-NHEJ) pathway that predominantly joins ends that lack homology (direct joints). However in C-NHEJ-deficient conditions, an alternative end-joining (A-EJ) pathway is left, which predominantly joins ends by using short homologies found in the proximity of broken ends (microhomology-based repair) [11] , [13] . The 3′RR is crucial for conventional CSR [6] , [7] but its mechanistic contribution remains enigmatic. The main conclusions drawn from knock-out mice are that the 3′RR plays a major role in promoting synapsis between S regions targeted by CSR [16] , and plays a partial role in promoting germline transcription of S regions initiating at I promoters [6] , [17] , [18] . Whether the chromatin structure of S regions or the process of their repair after CSR are also dependent from the 3′RR is currently unknown. The IgG 1 class displays a special status with regard to 3′RR mutations, since it was the only Ig class whose expression was preserved after the first reported partial 3′RR alterations or truncations [17] , [18] . Even after complete deletion of the 3′RR , while CSR to all other class-switched Ig was nearly abolished, residual low-level CSR to IgG 1 was maintained [6] . We thus now take advantage of this preserved IgG 1 switching in 3′RR -deficient mice to explore whether it reveals additional 3′RR -dependent mechanistic features during CSR. We report here that, even if some IgG 1 CSR still occurs, the 3′RR defect impacts the S γ1 acceptor region (rather than the donor S μ region) in multiple aspects that precede CSR. This includes alterations of epigenetic marks, germline transcription, R loop formation, paused RNA Pol II, AID targeting, and generation of DSBs. In contrast, once DSBs are generated, their repair is completely normal in 3′RR -deficient animals. Altogether, this study precisely maps the activity of the 3′RR at the early phases of CSR, until the generation of DSBs, and shows that it has no contribution in the process of DNA repair between synapsed broken ends. Deletion of the 3′RR impairs C μ - C γ1 CSR The IgH C γ1 gene has long been claimed to carry some specific regulatory elements and notably an upstream I γ1 enhancer [19] . While the IgH 3′RR is the major cis -element promoting synapsis between S regions and recruiting AID to the IgH locus, several previous descriptions of 3′RR disruptions in the mouse indicated some persistence of CSR to C γ1 [6] , [16] , [17] , [18] , and we thus decided to analyse in details the molecular features of this residual 3′RR -independent CSR. We confirmed that splenocytes from 3′RR -deficient mice showed a dramatically reduced ability to secrete IgG 1 in vitro in response to LPS+IL4 ( Fig. 1a ), which likely results from both decreased CSR in B-cells and the known defect of Ig secretion in plasma cells from such mice [6] . Parallel flow cytometry experiments evaluating membrane IgG 1 expression in B-cells confirmed that the deletion of the 3′RR did not abolish but reduced by >90% in vitro IgG 1 CSR ( Fig. 1b ). This strong but incomplete defect was also indicated by Southern blot experiments (full blots are included in the Supplementary Fig. 2 ) evaluating hybrid S μ - S γ1 junctions in 3′RR -deficient mice ( Fig. 1c ). Junctions were first amplified using a touch-down PCR followed with a nested PCR and revealed after hybridization with a 32 P-labelled probe. DNA from AID-deficient B-cells (devoid of any CSR) was used as germline control DNA. The IgG 1 CSR defect was also evidenced by real-time-PCR evaluation of post-switch IgG 1 transcripts ( Fig. 1d ). Finally, serum IgG 1 levels paralleled results obtained after in vitro stimulation ( Fig. 1e ) and confirmed that, altogether, the deletion of the 3′RR strongly but only partially blocks IgG 1 CSR. 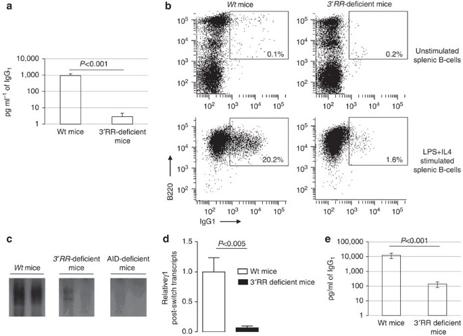Figure 1: Influence of the3’RRdeletion on IgG1CSR and secretion. (a) ELISA analysis of IgG1in supernatants of 3 days LPS+IL4 cultured B-cells. Data are the mean±s.e.m. of 8 experiments with 1 mouse (Mann–WhitneyU-test for significance). (b) B splenocytes ofwtand3′RR-deficient mice were isolated (upper panel) and stimulated with LPS+IL-4 for 3 days (lower panel). Cells were labelled with anti-B220-APC antibodies and anti-IgG1-FITC antibodies. Percentage of B220+IgG1+cells is reported in the gate. One representative experiment out of four (one mouse per experiment) is shown. (c) Southern blot analysis ofSμ-Cγ1junctions amplified by PCR and hybridized with a 5′Cγ1probe from 3 days LPS+IL4 stimulated splenocytes fromwt,3’RR-deficient mice and AID-deficient mice. DNA from AID-deficient B-cells (devoid of any CSR) was used as germline control DNA. Fifty nanograms and 20 ng of DNA were used for PCR experiments, respectively. One representative experiment out of four (one mouse per experiment) is shown. (d) Real-time PCR analysis of post switched IgG1transcripts in 3 days LPS+IL4 cultured B cells. Values were normalized toGapdhtranscripts. Data are the mean±s.e.m. of 8 to 11 independent experiments with one mouse (Mann–WhitneyU-test for significance). (e) ELISA analysis of IgG1in 12-week-old mice sera. Data are the mean±s.e.m. of 8 mice for each genotype (Mann–WhitneyU-test for significance). Figure 1: Influence of the 3’RR deletion on IgG 1 CSR and secretion. ( a ) ELISA analysis of IgG 1 in supernatants of 3 days LPS+IL4 cultured B-cells. Data are the mean±s.e.m. of 8 experiments with 1 mouse (Mann–Whitney U -test for significance). ( b ) B splenocytes of wt and 3′RR -deficient mice were isolated (upper panel) and stimulated with LPS+IL-4 for 3 days (lower panel). Cells were labelled with anti-B220-APC antibodies and anti-IgG 1 -FITC antibodies. Percentage of B220 + IgG 1 + cells is reported in the gate. One representative experiment out of four (one mouse per experiment) is shown. ( c ) Southern blot analysis of S μ - C γ1 junctions amplified by PCR and hybridized with a 5′ C γ1 probe from 3 days LPS+IL4 stimulated splenocytes from wt , 3’RR -deficient mice and AID-deficient mice. DNA from AID-deficient B-cells (devoid of any CSR) was used as germline control DNA. Fifty nanograms and 20 ng of DNA were used for PCR experiments, respectively. One representative experiment out of four (one mouse per experiment) is shown. ( d ) Real-time PCR analysis of post switched IgG 1 transcripts in 3 days LPS+IL4 cultured B cells. Values were normalized to Gapdh transcripts. Data are the mean±s.e.m. of 8 to 11 independent experiments with one mouse (Mann–Whitney U -test for significance). ( e ) ELISA analysis of IgG 1 in 12-week-old mice sera. Data are the mean±s.e.m. of 8 mice for each genotype (Mann–Whitney U -test for significance). Full size image Intra S μ deletion in 3′RR -deficient B cells It could be argued that the few S μ - S γ1 joints found in 3′RR -deficient B-cells mask a defect in end-joining that would result in aborted CSR (and, therefore, no joint to analyse). To test this hypothesis we analysed intra S μ deletions that frequently happen in mature B-cells during CSR [20] . By using a PCR amplifying the whole S μ region followed by Southern blotting, we checked that B-cell stimulation yielded fragments of different lengths corresponding to partial deletion of S μ during CSR. A similar pattern was found for both wt mice and 3′RR -deficient mice ( Fig. 2a ), eliminating any global defect in end joining in 3′RR -deficient mice and also showing that S μ is efficiently targeted by the CSR machinery in stimulated 3′RR -deficient B cells. 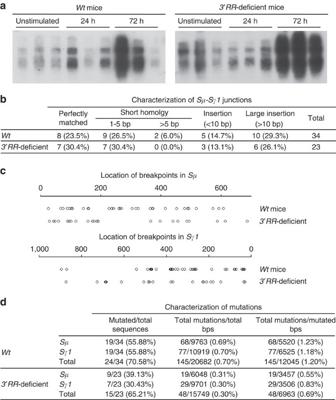Figure 2: Influence of the3′RRdeletion on diversity and mutations ofSμ-Sγ1junctions. (a) IntraSμdeletion in3’RR-deficient B cells. Splenocytes were LPS+IL4 stimulated for 24 or 72 h. PCR amplification of the wholeSμ region was followed by Southern blotting for detection of fragments of different length, more abundantly after B-cell stimulation, corresponding to partial deletion ofSμduring CSR. A similar pattern is found forwtand3′RR-deficient mice. Results from three mice out of six for each genotype are reported. (b) B splenocytes were stimulated with LPS+IL-4 to generateCμ-Cγ1CSR.Sμ-Sγ1junctions were cloned and sequenced. Percentage of junctions with insertion and junctional microhomology are indicated. Data are pooled from 6 independent experiments with 1 mouse per experiment forwtmice and 10 independent experiments with 1 mouse for3’RR-deficient mice. All junctions are reported in theSupplementary Table 1. (c) Location ofSμ-Sγ1breaks duringin vitroIgG1CSR (6wtmice and 103’RR-deficient mice; same junctions and mice as in (a). (d) Number of mutations and mutation frequency in the donor region (Sμ) and the acceptor region (Sγ1) duringCμ-Cγ1CSR. 34wtjunctions (data are pooled from 6 independent experiments with 1 mouse per experiment) and 233′RR-deficient junctions (data are pooled from 10 independent experiments with 1 mouse per experiment; same junctions and mice as in (b,c)). Figure 2: Influence of the 3′RR deletion on diversity and mutations of S μ - S γ1 junctions. ( a ) Intra S μ deletion in 3’RR -deficient B cells. Splenocytes were LPS+IL4 stimulated for 24 or 72 h. PCR amplification of the whole S μ region was followed by Southern blotting for detection of fragments of different length, more abundantly after B-cell stimulation, corresponding to partial deletion of S μ during CSR. A similar pattern is found for wt and 3′RR -deficient mice. Results from three mice out of six for each genotype are reported. ( b ) B splenocytes were stimulated with LPS+IL-4 to generate C μ - C γ1 CSR. S μ - S γ1 junctions were cloned and sequenced. Percentage of junctions with insertion and junctional microhomology are indicated. Data are pooled from 6 independent experiments with 1 mouse per experiment for wt mice and 10 independent experiments with 1 mouse for 3’RR -deficient mice. All junctions are reported in the Supplementary Table 1 . ( c ) Location of S μ - S γ1 breaks during in vitro IgG 1 CSR (6 wt mice and 10 3’RR -deficient mice; same junctions and mice as in ( a ). ( d ) Number of mutations and mutation frequency in the donor region ( S μ ) and the acceptor region ( S γ1 ) during C μ - C γ1 CSR. 34 wt junctions (data are pooled from 6 independent experiments with 1 mouse per experiment) and 23 3′RR -deficient junctions (data are pooled from 10 independent experiments with 1 mouse per experiment; same junctions and mice as in ( b , c )). Full size image Analysis of S -junctions in residual C μ - C γ1 CSR To analyse S -junctions, the amplified PCR S μ - S γ1 fragments were cloned, sequenced and aligned with the germline S μ and S γ1 sequences ( Fig. 2b and Supplementary Table 2 ). The deletion of the 3′RR had no effect on the structure of S junctions with regards to the relative amounts of direct joints, the frequency and length of microhomologies and the frequency of DNA insertion at the junction and of complex junctions. This suggests that beyond the AID targeting, DSBs and S μ - S γ1 synapsis steps, the late CSR resolution step is completely 3′RR -independent and remains unbiased in the choice between either the C-NHEJ or the A-EJ pathways for repairing broken DNA ends. We then analysed whether the absence of the 3′RR enhancers affected the position of the S μ and S γ1 breakpoints, which might indicate changes in the targeting or the synapsis of these regions. S μ breakpoints appeared unaltered, with the vast majority of them located in the 5′ part (0–600 bp) of S μ ( Fig. 3 ): 97% (33/34) and 91% (21/23) for wt and 3′RR -deficient mice, respectively ( Fig. 2c ). The 3′RR deletion by contrast affected the location of S γ1 breakpoints since 94% (32/34) of breaks cloned from wt cells were located in the 3′ part (0–480 bp) of S γ1 , while only 65% (15/23) were included in this segment in 3′RR -deficient cells. The pattern of AID targeting that initiates the formation of DSBs is thus 3′RR -independent within S μ but partially 3′RR -dependent within S γ1 . The increased representation of DNA breaks in the 3′ part of S γ1 (>480 bp) was not linked to the presence of microhomologous sequences: 2/4 and 6/11 direct junctions for wt and 3′RR -deficient mice, respectively. We conclude that the recombination of S μ with S γ1 in 3′RR -deficient B cells does not depend on the presence of microhomologous sequences and that the 3′RR is not involve in the resolution of CSR nor in the choice between C-NHEJ and A-EJ pathways. 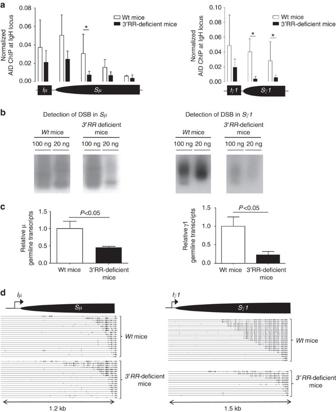Figure 3: AID and CSR in3′RR-deficient mice. (a) AID ChIP assays were performed with splenic B cells from3’RR-deficient andwtmice. Cells were stimulated with LPS+IL-4 for 2 days. Background signals from mock samples with irrelevant antibody were subtracted. Values were normalized to the total input DNA. Data are the mean±s.e.m. of six independent experiments with two mice. *P<0.05 (Mann–WhitneyU-test). (b) Ligation-mediated PCR. Splenic B cells were stimulated with LPS+IL-4 for 2 days. Genomic DNA fromwtand3′RR-deficient mice were treated with T4 DNA polymerase (T4 Pol), ligated with T4 DNA ligase and probed for double-stranded breaks inSμandSγ1by semi-nested PCR. Reactions with 100 and 20 ng of DNA are shown. Data are representative of four experiments each with one mouse per genotype. (c) Real-time PCR analysis ofIμ-CμandIγ1-Cγ1transcripts in 3 days LPS+IL4 cultured B cells. Values were normalized toGapdhtranscripts. Data are the mean±s.e.m. of 8 to 11 independent experiments with 1 mouse (Mann–WhitneyU-test for significance). (d) Detection of R loops inSμandSγ1. Cells were stimulated with LPS+IL-4 for 2 days. DNA was extracted, bisulfited, treated and sequenced to detect single strand inSμandSγ1regions. Each long line represents an independent sequence. The small vertical bars on each line indicate a C on the sequence converted to a T, indicating that the sequence was in a single-strand conformation. Pooled results from six independent experiments each with one mouse per genotype. Figure 3: AID and CSR in 3′RR -deficient mice. ( a ) AID ChIP assays were performed with splenic B cells from 3’RR -deficient and wt mice. Cells were stimulated with LPS+IL-4 for 2 days. Background signals from mock samples with irrelevant antibody were subtracted. Values were normalized to the total input DNA. Data are the mean±s.e.m. of six independent experiments with two mice. * P <0.05 (Mann–Whitney U -test). ( b ) Ligation-mediated PCR. Splenic B cells were stimulated with LPS+IL-4 for 2 days. Genomic DNA from wt and 3′RR -deficient mice were treated with T4 DNA polymerase (T4 Pol), ligated with T4 DNA ligase and probed for double-stranded breaks in S μ and S γ1 by semi-nested PCR. Reactions with 100 and 20 ng of DNA are shown. Data are representative of four experiments each with one mouse per genotype. ( c ) Real-time PCR analysis of I μ - C μ and I γ1 - C γ1 transcripts in 3 days LPS+IL4 cultured B cells. Values were normalized to Gapdh transcripts. Data are the mean±s.e.m. of 8 to 11 independent experiments with 1 mouse (Mann–Whitney U -test for significance). ( d ) Detection of R loops in S μ and S γ1 . Cells were stimulated with LPS+IL-4 for 2 days. DNA was extracted, bisulfited, treated and sequenced to detect single strand in S μ and S γ1 regions. Each long line represents an independent sequence. The small vertical bars on each line indicate a C on the sequence converted to a T, indicating that the sequence was in a single-strand conformation. Pooled results from six independent experiments each with one mouse per genotype. Full size image Influence of the 3′RR on AID recruitment during C μ - C γ1 CSR Before the occurrence of DSBs, CSR is initiated by AID and the initial outcome of AID targeting can be the occurrence of base substitutions following cytidine deamination [12] , [14] , [15] , [21] . To gain an insight into this initial targeting, we analysed mutations in S regions and observed that both the S μ donor and S γ1 acceptor regions are less targeted by AID during IgG 1 CSR in 3′RR -deficient mice as compared with wt animals ( Fig. 2d ). This showed up with mutation rates falling at 55 and 30% of their wt levels for S μ and S γ1 , respectively. This observation suggests a lower recruitment of AID in S regions in 3′RR -deficient animals, which is indeed also indicated by ChIP experiments showing a significantly decreased AID loading at both the S μ and S γ1 regions (after 2 days LPS+IL4 in vitro stimulation) in 3′RR -deficient mice compared with wt mice ( Fig. 3a ). A crucial step of CSR is the processing of AID lesions into DSBs, as a specific feature of S regions [14] , [15] . Ligation-mediated PCR (LM-PCR, see Supplementary Fig. 1b ) was used to highlight DSBs in S μ and S γ1 . Thus, extracted genomic DNA was treated with T4 DNA polymerase yielding blunt DNA ends, then ligated with T4 DNA ligase with a double-strand anchor linker [22] . DSBs were detected by semi-nested PCR (primers targeting the linker sequence and a primer specific to S μ or S γ1 ) followed by hybridization with a 32 P-labelled probe. LM-PCR highlighted a small reduction of DSBs in S μ but a dramatic one in S γ1 in 3′RR -deficient mice compared with wt mice ( Fig. 3b ; full blots are included in the Supplementary Fig. 2 ). Impaired induction of DNA lesions during CSR was suggested in patients to influence end joining [23] . It is obviously not the case in 3′RR -deficient mice. The substrate for AID is single-strand DNA (ssDNA) which is generated by germline transcription of S regions and Ig constant regions on both the transcribed and non-transcribed strands. Real-time PCR analysis only indicated a partial reduction of I μ - C μ and I γ1 - C γ 1 transcripts in 3′RR -deficient mice ( Fig. 3c ), as previously suggested by semi-quantitative PCR [6] . This shows that the 3′RR does not promote CSR only by fostering germline transcription. Transcription through S regions generates R loops in which the RNA stably hybridizes to the template strands, displacing the non-template strand as ssDNA [14] , [15] . For R loops experiments (see Supplementary Fig. 1c ), extracted DNA was treated with bisulfite. Thus, only C located on ssDNA patchs (that is, in R loops) could be converted in U. Bisulfite-treated DNA was then amplified by PCR and sequenced to detect R loops in S μ and S γ1 regions. As shown in Fig. 3d , the formation of R loops was markedly altered in S γ1 region but not in S μ region of 3′RR -deficient mice (each long line represents an independent sequence and the small vertical bars on each line indicate a C on the sequence converted to a T, indicating that the sequence was in a single-strand conformation). R loops in the S μ region appear to be even longer in 3′RR -deficient mice, a result that might be taken as an indication of the reduced CSR efficiency due to the reduced S γ1 CSR priming. AID was shown to be in a complex with RNA Pol II (Pol II P-ser2) and paused RNA Pol II (Pol II P-ser5) [24] . ChIP experiments showed a weak decrease in the load of RNA Pol II (but not paused RNA Pol II) in the I μ – S μ – C μ region ( Fig. 4a,b ). By contrast, 3′RR -deficient cells showed dramatically decreased binding of RNA Pol II and paused RNA Pol II throughout the P γ1 - I γ1 - S γ1 - C γ1 region ( Fig. 4a,b ). Collectively, our data indicated that the 3′RR is of key importance for the regulation, in S γ1 region, of RNA Pol II recruitment, transcriptional activity and pausing, that is known prerequisites of AID recruitments. The lower accumulation of AID in the S γ1 region of 3′RR -deficient mice translates into lower amounts of DSBs and thus reduced efficiency of IgG 1 CSR. Lower S γ1 RNA Pol II targeting and I γ1 - C γ1 germline transcription are also in agreement with reduced length of S γ1 R loops. Of interest, the S μ donor region was markedly less affected by the 3′RR deletion than the S γ1 acceptor region, suggesting that S μ is the less 3′RR -dependent S region of the IgH locus at both the level of transcription and AID targeting. Reduced S μ - S γ1 CSR in 3′RR -deficient mice thus mostly involves decreased accessibility and less frequent DSBs in the acceptor S γ1 than in the donor S μ region. 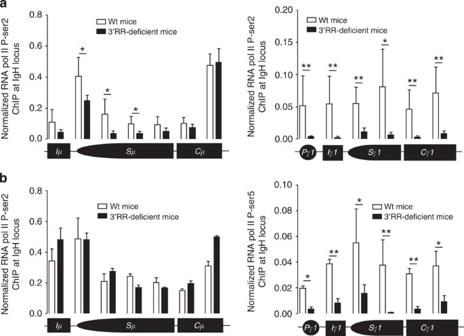Figure 4: RNA Pol II during CSR in3′RR-deficient mice. ChIP assays were performed with splenic B cells from3′RR-deficient andwtmice. Cells were stimulated with LPS+IL-4 for 2 days. RNA Pol II P-ser 2 (a). RNA Pol II P-ser 5 (b). Background signals from mock samples with irrelevant antibody were subtracted. Values were normalized to the total input DNA. Data are the mean±s.e.m. of three experiments with two mice for each genotype. *P<0.05 and **P<0.01 (Mann–WhitneyU-test). Figure 4: RNA Pol II during CSR in 3′RR -deficient mice. ChIP assays were performed with splenic B cells from 3′RR -deficient and wt mice. Cells were stimulated with LPS+IL-4 for 2 days. RNA Pol II P-ser 2 ( a ). RNA Pol II P-ser 5 ( b ). Background signals from mock samples with irrelevant antibody were subtracted. Values were normalized to the total input DNA. Data are the mean±s.e.m. of three experiments with two mice for each genotype. * P <0.05 and ** P <0.01 (Mann–Whitney U -test). Full size image Chromatin remodelling in the absence of the IgH 3′RR Histone H3 and H4 modifications (acetylation and methylation) are implicated in the targeting of the CSR machinery (including AID and RNA Pol II) to S regions primed for CSR [25] , [26] , [27] , [28] . Altogether with DNA transcription, this remodelling of chromatin in S regions constitutes a hallmark of the accessibility to CSR factors. As shown in Fig. 5 , except for acetylated lysine 9 in histone H3 (H3K9ac), levels of H3 acetylation (H3ac), H4 acetylation (H4ac) and trimethylated lysine 4 in histone H3 (H3K4me3) were not affected by the deletion of 3′RR enhancers in the I μ - S μ - C μ region during IgG 1 CSR induced by LPS+IL4 stimulation. In contrast, H3ac, H3K4me3 and H3K9ac were dramatically lowered in the P γ1 - I γ1 - S γ1 - C γ1 region (while H4ac was unchanged) ( Fig. 5 ). Interestingly, the H3K4me3 and H3K9ac marks are required for efficient CSR and further AID recruitment [27] , [28] . As reported above for AID and RNA Pol II, this study of the epigenetic marks required for CSR shows that the 3′RR mostly acts on accessibility of the acceptor S γ1 rather than the donor S μ region during S μ - S γ1 CSR. This suggests that a reduction in histone acetylation is the most upstream defect after 3′RR deletion. The levels of histone acetylation are reversibly controlled by the balanced counteraction of histone acetyltransferases (HATs) and histone deacetylases (HDACs). Although HDAC inhibitor treatment have been used to reverse the heterochromatin silencing of Ig minigenes [29] , these drugs are potent inhibitors of the 3′RR in B cells. Thus, treatment of B cells with the HDAC inhibitor trichostatin A represses IgH gene transcription, CSR and Ig synthesis in B splenocytes [30] . We confirmed that IgG 1 CSR was strongly decreased in activated B-cells treated with trichostatin A, valproic acid or SAHA; three HDAC inhibitors ( Supplementary Fig. 3 ). Therefore, ChIP assays of epigenetic marks should be preferred over HDAC inhibitor treatments to study CSR in the IgH locus. How 3′ RR recruits histone acetyltransferases (if any) remains an open question. Studies suggested that levels of histone acetylation in the IgH locus are predominantly controlled by HDACs, but that the various HDACs might have opposite effects. ChIP experiments reported HDAC1 recruitment by the central hs1,2 enhancer of the 3′RR [30] and IgH transcription decreased in HDAC1-deficient chicken B cells [31] . By contrast, HDAC2 inhibited transcription and recombinational activities at the IgH locus [31] . 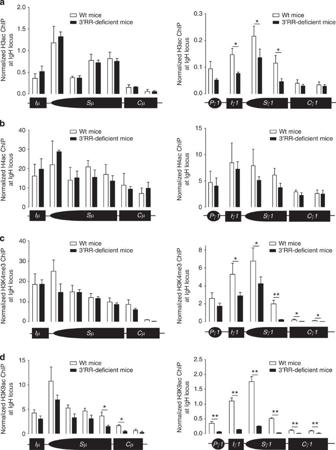Figure 5: Epigenetic marks (H3ac, H4ac, H3K4me3 and H3K9ac) inSμandSγ1during IgG1CSR in3’RR-deficient mice. ChIP assays were performed with splenic B-cells from3’RR-deficient andwtmice. Cells were stimulated with LPS+IL-4 for 2 days. Background signals from mock samples with irrelevant antibody were subtracted. Values were normalized to the total input DNA. Data are the mean±s.e.m. of three (for3’RR-deficient mice) and six (forwtmice) independent experiments with two mice (Mann–WhitneyU-test for significance). Figure 5: Epigenetic marks (H3ac, H4ac, H3K4me3 and H3K9ac) in S μ and S γ1 during IgG 1 CSR in 3’RR -deficient mice. ChIP assays were performed with splenic B-cells from 3’RR -deficient and wt mice. Cells were stimulated with LPS+IL-4 for 2 days. Background signals from mock samples with irrelevant antibody were subtracted. Values were normalized to the total input DNA. Data are the mean±s.e.m. of three (for 3’RR -deficient mice) and six (for wt mice) independent experiments with two mice (Mann–Whitney U -test for significance). Full size image Effect of the 3′RR on S γ3 , 2b , ɛ acceptor regions during CSR Other CSR-related S acceptor regions are located all along the IgH locus ( Supplementary Fig. 1a ). As previously reported the 3′RR not only interacts with S γ1 but also other S regions including S γ3 , S γ2b and S ɛ [16] . We evaluated what happens for S γ3 , S γ2b and S ɛ after appropriate in vitro CSR stimulations. Similarly to S γ1 , we found a dramatic decrease of AID, pol II, paused pol II recruitments and H3K9ac/H3K4me3 levels in S γ3 , S γ2b and S ɛ in B cells of 3′RR -deficient mice compared with wt mice ( Fig. 6 ). Taken altogether, these results reveal a similar mechanistic role of the 3′RR on S acceptor regions during CSR and confirm its key role on Ig production [6] , [7] . 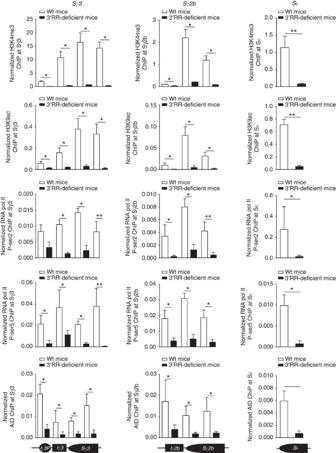Figure 6: Epigenetic marks, AID and pol II recruitments inSγ3,Sγ2bandSɛduring CSR in3′RR-deficient mice. ChIP assays were performed with splenic B-cells from3′RR-deficient andwtmice. Cells were stimulated with LPS for 2 days forSγ3andSγ2b. Cells were stimulated with LPS±IL4 for 2 days forSɛ. Background signals from mock samples with irrelevant antibody were subtracted. Values were normalized to the total input DNA. Data are the mean±s.e.m. of three to six independent experiments with two mice for each genotype (Mann–WhitneyU-test for significance). Figure 6: Epigenetic marks, AID and pol II recruitments in S γ3 , S γ2b and S ɛ during CSR in 3′RR -deficient mice. ChIP assays were performed with splenic B-cells from 3′RR -deficient and wt mice. Cells were stimulated with LPS for 2 days for S γ3 and S γ2b . Cells were stimulated with LPS±IL4 for 2 days for S ɛ . Background signals from mock samples with irrelevant antibody were subtracted. Values were normalized to the total input DNA. Data are the mean±s.e.m. of three to six independent experiments with two mice for each genotype (Mann–Whitney U -test for significance). Full size image Transcriptional profiles of 3′RR -deficient B cells Transcriptional profiles evidenced differences between splenic B cells of 3′RR -deficient and wt mice ( Supplementary Table 3 ). Several genes implicated in interferon-related functions, inflammation, cell trafficking and B-cell homing were affected in resting B splenocytes of 3′RR -deficient mice (accession number GSE45230 , Gene Expression Omnibus database). Since the cis -regulatory element 3′RR is not expected to modulate genes outside the IgH locus, these differences rather involve the recently reported decreased accumulation of marginal zone B cells in 3′RR -deficient mice [32] . Accordingly, functions of the affected genes fit well with roles of marginal zone B cells in infection, inflammation and immunity. After 3 days LPS+IL4 stimulation, some genes were differentially affected ( Supplementary Table 4 ). In relations with the marked influence of the 3′RR on histone modifications during CSR, inhibitors of histone acetyltransferase ( Anp32a, Tle1 ), histone demethylase ( Eco1 ) and histone deacetylase ( Cbl-b ) are overexpressed in stimulated 3′RR -deficient splenocytes as compared with wt cells. In agreement with lower frequency of DSB, genes implicated in DSB detection and reparation were either downregulated ( Atm , Lig4 ) or upregulated ( Parp-3 , H2afx , Ino80 and Esco1 ). While a direct effect of the cis -regulatory 3′RR on genes located outside of the IgH locus is unlikely, gene variations rather appear related to incomplete CSR. Strikingly, RNA sequencing analysis did not identify similar gene variation in LPS+IL4 stimulated AID-deficient splenic B cells (thus lacking any AID-mediated DNA lesions) compared with wt [32] . This suggests that genes implicated in CSR repair are highly regulated and only transiently expressed in wt cells in response to DSBs in S μ and S γ1 . AID-deficient and 3′RR -deficient mice carry CSR defect by completely different mechanisms, with, respectively, a lack of DSBs (both on S μ and S γ1 ) or a biased occurrence of DSBs (normally targeting S μ but not S γ1 ). Gene variations in 3′RR -deficient mice are thus likely not reflecting simply the lack of CSR per se , but rather the status of cells poised for CSR, some of them displaying DSBs in S μ , and unable to efficiently repair these DSBs through long-range recombination with a distant acceptor region. In conclusion, we favour the hypothesis that persistent DNA damage in S μ would increase the expression of genes involved in DNA-repair in 3′RR -deficient B cells. miRNA analysis in 3′RR -deficient B cells If the hypothesis that persistent DNA damages in S μ affect gene expression profiles in 3′RR -deficient B-cells is correct, variation might also be evidenced at the miRNA level. To further explore how the 3′RR deletion impacts the activation of B cells during CSR, we measured the expression of a panel of 84 miRNA known to be involved in B-cell development and activation. We investigated miRNA in LPS+IL4 stimulated AID-deficient splenic B-cells and found 18 downregulated miRNA and 2 up-regulated miRNA compared with wt mice ( Supplementary Fig. 4 ). In contrast, 0 miRNA were downregulated and 11 miRNA were up-regulated in 3′RR -deficient mice ( Supplementary Fig. 4 ) compared with wt mice. Up-regulated miRNA in 3′RR -deficient mice have hundreds of predicted targets, including Atm , Ssb1 , Ino80 , Exo1 , Smarcd1 , Dclre1b and Atmin , which have been shown to regulate DSB resection and homologous recombination [33] , [34] , [35] , [36] , [37] , [38] , and histone modifying enzymes Hdac9 and Esco1 . Interestingly, HDAC9 is required for DSB reparation by homologous reparation [39] , and its deletion affects antibody secretion [40] . Altogether, this might inhibit A-EJ, by downregulating gene implicated in microhomology based DSB repair ( Atm , Atmin , Ssb1 and Hdac9 ), and to favour NHEJ by upregulating Parp-3 [41] , and Esco1 , which influence the interaction between cohesion complex and DNA required for efficient NHEJ [42] , [43] . A-EJ has been shown to facilitate oncogenic translocations to IgH locus and to be less restricted to intrachromosomal joining than NHEJ [20] . This might be a protective mechanism limiting oncogenic translation to S μ , in which DSBs appear quite frequently while there are few in downstream acceptor regions. In parallel, LM-PCR did not show accumulation of DSBs in S μ in 3′RR -deficient mice, despite the lack of complete CSR, suggesting that intraswitch junctions, which occur normally, are the usual mean that can be used by B cells to resolve abortive CSR issues. Finally, taken altogether results of miRNA analysis reinforce the hypothesis that the prolonged presence of DNA damage in S μ would affect gene expression in 3′RR -deficient B-cells rather that the hypothetical loss of 3′RR trans-interactions with these genes in the nuclei. In the present study we show that the 3′RR promotes IgG 1 CSR not only by fostering germline transcription but also histone modifications (especially H3K4me3 and H3K9ac), formation of R loops, loading and pausing of RNA Pol II, AID recruitment and finally generation of DSBs in the S γ1 region, indicating that the 3′RR enhancers act as soon as these initial steps of the CSR process. In contrast to the S γ1 region, S μ appears as more or less 3′RR -independent, suggesting that other regulatory elements are required for its CSR formatting. In a previous study Wuerffel et al . [16] demonstrated with 3C assay and hs3b/hs4-deficient mice that the 3′RR interacted with the S γ1 region whereas S μ was closely associated with E μ . Moreover the non conventional IgD CSR (between S μ and a S δ -like region) occurs independently of the 3′RR [7] . Our study thus validates at the DNA level the hypothesis that during CSR, the 3′RR especially targets the S acceptor region rather than the S μ donor region. Although the Eμ enhancer could be proposed to support S μ accessibility when the 3′RR is deleted, it is noteworthy that it is not itself mandatory for CSR [3] . The 3′RR -independence of S μ is also somehow striking comparing with the known 3′RR -dependence of pV H promoters and rearranged VDJ regions with regards to AID recruitment and SHM [8] . Finally, that S γ1 accessibility to CSR is only partly altered in the absence of the 3′RR allowed to study residual CSR junctions, showing that their molecular features were indiscernible from those of wt junctions studied in parallel. This suggests that the 3′RR contribution to CSR is restricted to the early steps of accessibility, AID recruitment and synapsis of target regions, but with no role in the repair and final resolution of CSR. Our analysis also showed that B-cells are able to transiently modify their transcriptome and miRNome during CSR to foster rapid and precise repair of DSBs, thus diminishing the risk of potentially oncogenic translocation. Mice The 129 wt mice (from Charles Rivers Laboratories, France) and 3′RR -deficient mice (from UMR CNRS 7276, Limoges, France; in a 129 background) were used. Mice of 2-3 months old (male and female) were investigated. Our research has been approved by our local ethics committee review board (Comité Régional d'Ethique sur l'Expérimentation Animale du Limousin, Limoges, France) and carried according the European guidelines for animal experimentation. Spleen cell cultures for CSR Single-cell suspensions of CD43 − spleen cells were cultured 3 days at 1 × 10 6 cells ml −1 in RPMI 1640 with 10% fetal calf serum, 5 μg ml −1 LPS with or without 20 ng ml −1 IL-4 (PeproTech, Rocky Hill, NJ) [6] . Cell cytometry analysis Single-cell suspensions of cultured B cells were incubated with anti-B220-SpectralRed (PC5)-labelled antibodies (Biolegends, ref:103210, 10 μg ml −1 final) and anti-IgG 1 -fluorescein-isothiocyanate (FITC)-labelled antibodies (Southern Biotechnologies, ref:107002, 10 μg ml −1 final) and analysed on a Fortessa LSR2 (Beckton-Dickinson) [44] , [45] . Cloning and sequencing of S μ -S γ1 junctions Three days in vitro stimulated splenocytes were harvested and DNA was extracted for investigation of S μ - S γ1 junctions. Junctions were studied using a touch-down PCR followed with a nested PCR using the following parameters: Touch-down PCR: Forward primer 5′- AGAGACCTGCAGTTGAG GCC -3′ and backward primer 5- AGGATGTCCACCCTCACCCAGGC -3′ (1 cycle, 98 °C for 30 s; 2 cycles, 98 °C for 10 s, 69 °C for 30 s, 72 °C for 90 s; 2 cycles, 98 °C for 10 s, 67 °C for 30 s, 72 °C for 90 s; 2 cycles, 98 °C for 10 s, 65 °C for 30 s, 72 °C for 90 s; 25 cycles, 98 °C for 10 s, 60 °C for 30 s, 72 °C for 90 s 1 cycle, 72 °C for 7 min). Nested PCR: Forward primer 5′- CCAGCCACAGTAATGACCCAG -3′ and backward primer 5′- TTGTTATCCCCCATCCTGTCACCT -3′ (1 cycle, 98 °C for 30 s; 35 cycles, 98 °C for 10 s, 65 °C for 30 s, 72 °C for 90 s; 1 cycle, 72 °C for 7 min). The PCR products were cloned into the Zero Blunt Topo PCR cloning (Invitrogen). Plasmids were isolated using the NucleoSpin kit (Macherey-Nagel Eurl) and sequenced using an automated laser fluorescent ANA ABI-PRISM sequencer (Perkin-Elmer). Southern blotting of C μ -C γ1 junctions S μ - S γ1 junctions amplified as previously described were subjected to 1% agarose gel electrophoresis, and transferred overnight on a positively charged Nylon hybridization membrane (MP Biomedicals). A 507bp probe was amplified using the following primers: Forward primer 5′- GGCAGATTAGAATGAATGCACCTG-3′ , backward primer 5′- TTGTTATCCCCCATCCTGTCACCT and 32 P-labelled using Amersham Rediprime II Random Prime Labelling System (GE Healthcare) according to the manufacturer protocol. The membranes were saturated with salmon sperm DNA (4mgml −1 ) and incubated with the labelled probe overnight at 42°C. Membrane were then washed for 15 minutes twice at room temperature in 2X SSC buffer+0.1% SDS, then 5 minutes at 52°C in 0.1X SSC+0.5% SDS. Membranes were autoradiographed on X50 hyperfilm MP (GE Healthcare) at −80°C for 6 hours and revealed using Carestream Kodak autoradiography GBX developer and fixer (Sigma Aldrich). IgG 1 Elisa assays Blood samples were recovered from 12 weeks-old transgenic mice and wt controls. Serum samples were recovered by centrifugation and stored at −20 °C until used. B splenocytes were cultured for 3 days with LPS+IL4. At day 3, 1 × 10 6 cells were cultured for 24 h in growth medium without LPS+IL4. Culture supernatants were recovered and stored at −20 °C until used. Culture supernatants and sera were analysed for the presence of IgG 1 by ELISA [6] , [44] , [45] . ELISA assays were performed in polycarbonate 96 multiwell plates, coated overnight at 4 °C (100 μl per well) with 2 μg ml −1 IgG 1 (Cell Lab, ref:731863) in 0.05 M Na 2 CO 3 buffer. After three successive washing steps in phosphate-buffered saline (PBS) buffer, a blocking step was performed (3% bovine serum albumin (BSA) in PBS) for 30 min at 37 °C. After three washing steps, 50 μl of sera (first diluted to 1:50), supernatants or standard IgG 1 (Beckman Coulter, ref:731907, 1 mg ml −1 , first diluted to 1:50) were diluted into successive wells in 1% BSA/PBS buffer and incubated for 2 h at 37 °C. After three washing steps, 100 μl per well of 1 μg ml −1 AP-conjugated goat anti-mouse IgG 1 (Southern Biotechnologies, ref: 1070041) were incubated for 2 h at 37 °C. After washing, AP activity was assayed on 1 mg ml −1 AP substrate, and blocked with addition of 3 M NaOH. Optic density was then measured at 400 nm. Quantitative PCR of I γ1 -C γ1 and I μ -C γ1 transcripts Two days in vitro stimulated splenocytes were collected and RNA was extracted for investigation of I γ1 - C γ1 transcripts. RNA and cDNA were prepared using standard techniques. Quantitative PCR was performed using power SYBR green (Applied Biosystems): I γ1 forward primer: 5′- GGCCCTTCC AGATCTTTGAG -3′; C γ1 reverse primer: 5′- ATGGAGTTAGTTTGGGCAGCA -3′. I μ forward primer: 5′- ACCTGGGAATGTATGGTTGTGGCTT -3′. C μ reverse primer 5′- TCTGAACCTTCAAGGATGCTCTTG -3′. I γ1 - C γ1 and I μ - C γ1 transcripts were normalized to Gapdh transcripts (reference Mm99999915-g1). ChIP experiments Splenic B cells were purified by CD43 magnetic cell sorting from nonimmunized mice and cultured in vitro with 5 μg ml −1 LPS with or without 20 ng ml −1 IL4 for 2 days. ChIP experiments were done essentially as previously described [8] . In brief, 3 × 10 7 stimulated B cells were cross-linked at 37 °C for 15 min in 15 ml PBS with 1% formaldehyde. The reaction was quenched with 0.125 M glycine. After lysis, chromatin was sonicated to 0.5–1 kb using a Vibracell 75043 (Thermo Fisher Scientific). After dilution in ChIP buffer (0.01% SDS, 1.1% Triton X-100, 1.2 mM EDTA, 16.7 mM Tris-HCl, pH 8.1, and 167 mM NaCl), chromatin was precleared by rotating for 2 h at 4 °C with 100 μl of 50% protein A/G slurry (0.2 mg ml −1 sheared salmon sperm DNA, 0.5 mg ml −1 BSA, and 50% protein A/G; Sigma). 0.3−0.5 × 10 6 cell equivalents were saved as input, and 3−5 × 10 6 cell equivalents were incubated overnight with specific or control antibodies. Immune complexes were precipitated by the addition of protein A/G. Cross-linking was reversed by overnight incubation (70 °C) in TE buffer with 0.02% SDS and chromatin was phenol/chloroform extracted. PCR primers used for Q-PCR are detailed in the Supplementary Table 2 . The following antibodies were used: anti-H3K4me3 (Millipore, 07-473), anti-H3K9ac (Millipore, 06-942), anti-H3ac (Millipore, 06-599), anti-H4ac (Millipore, 06-866), anti-RNA Pol II P-ser2 (Abcam, ab5095) and anti-RNA Pol II P-ser 5 (Abcam, ab5131). Anti-AID antibodies were kindly provided by Dr P. Gearhart. Ligation-mediated PCR LM-PCR was used to highlight the presence of DSBs in S μ and S γ1 . LM-PCR experiments were schematized in the Supplementary Fig. 1b . Splenocytes were stimulated with LPS+IL4 for 2 days. Genomic DNA was extracted and treated with T4 DNA polymerase which trims back 3′overhangs while ‘filling in’ 3′-recessed ends, thereby yielding blunt 5′-phosphorylated DNA ends. DNA was then ligated with T4 DNA ligase with the double-strand anchor linker BW [22] . DSBs were detected by semi-nested LM-PCR using BW1 primer targeting the BW linker sequence and a primer specific to S μ or S γ1 . DSB were studied after hybridization with 32 P-labelled probes located on S μ and S γ1 , respectively. R loops R loops were analysed using bisulfite conversion of single-strand DNA [46] . R loop experiments were schematized in the Supplementary Fig. 1c . Splenic B-cells from wt and 3′RR -deficient mice were stimulated in vitro with 5 μg ml −1 LPS and 20 ng ml −1 IL4 for 2 days. DNA was extracted and purified using Phase Lock gel (5 Prime), and digested with EcoRI (New England Biolabs) for 8 h. DNA was bisulfite converted using the EpiMark Bisulfite Conversion Kit (New England Biolabs). Five micrograms were incubated in Bisulfite mix at 37 °C for 15 h. Converted DNA was then desulfonated and purified according to the manufacturer protocol, and resuspended in 60 μl H 2 O. We made touch-down PCR reaction (One Taq Hot start DNA polymerase, NEB) using a forward native primer and a reverse primer designed to match the converted sequence. For S μ : forward primer 5′- GCTGCTCTTAAAGCTTGT AAACTGTTTCT -3′ and backward primer 5- CTCACCCCATCTCAACTACTCCAAAA TAA -3′; (1 cycle, 94 °C for 30 s; 3 cycles, 94 °C for 15 s, 56 °C for 30 s, 68 °C for 120 s; 3 cycles, 94 °C for 15 s, 55 °C for 30 s, 68 °C for 120 s; 3 cycles, 94 °C for 15 s, 54 °C for 30 s, 68 °C for 120 s; 25 cycles, 94 °C for 15 s, 53 °C for 30 s, 68 °C for 120 s; 1 cycle, 68° for 5 min). For S γ1 : forward primer 5′- TTCCAGATCTTTGAGTCATCCTATC -3′ and backward primer 5- CACCCATCAACTCTA ACCATATAATATTTACTC -3′; (1 cycle, 94 °C for 30 s; 3 cycles, 94 °C for 15 s, 52 °C for 30 s, 68 °C for 120 s; 3 cycles, 94 °C for 15 s, 51 °C for 30 s, 68 °C for 120 s; 3 cycles, 94 °C for 15 s, 50 °C for 30 s, 68 °C for 120 s; 25 cycles, 94 °C for 15 s, 49 °C for 30 s, 68 °C for 120 s; 1 cycle, 68° for 5 min). The PCR products were cloned and sequenced as described for S μ - S γ1 junctions. Transcriptome analysis mRNA was extracted from B220 + splenic B-cells of 3′RR -deficient mice and wt mice before and after 3 days LPS+IL4 stimulation. Microarray experiments were done in ‘Nice - Sophia Antipolis Microarray Facility’ (France). Statistical analysis was made with the Bioconductor open source software, particularly its Limma package [47] , [48] , [49] , [50] . The microarray data presented in this article have been submitted to the Gene Expression Omnibus database ( www.ncbi.nlm.nih.gov/geo/ ) under the accession numbers GSE45230 . miRNA analysis Splenic B cells from wt , AID-deficient mice and 3′RR -deficient mice were stimulated in vitro with 5 μg ml −1 LPS and 20 ng ml −1 IL4 for 2 days, and total RNA was extracted. cDNA was prepared using QIAGEN miScript II RT kit, and expression of a panel of 84 miRNA was determined using QIAGEN miScript miRNA PCR Array Mouse T-Cell and B-Cell activation, according to the manufacturer’s protocol. miRNA targets predictions were made using the http://mirdb.org/ website [51] . How to cite this article: Saintamand, A. et al . Elucidation of IgH 3′ region regulatory role during class switch recombination via germline deletion. Nat. Commun. 6:7084 doi: 10.1038/ncomms8084 (2015).